Porous materials with pre-designed single-molecule traps for CO2selective adsorption Despite tremendous efforts, precise control in the synthesis of porous materials with pre-designed pore properties for desired applications remains challenging. Newly emerged porous metal-organic materials, such as metal-organic polyhedra and metal-organic frameworks, are amenable to design and property tuning, enabling precise control of functionality by accurate design of structures at the molecular level. Here we propose and validate, both experimentally and computationally, a precisely designed cavity, termed a ‘single-molecule trap’, with the desired size and properties suitable for trapping target CO 2 molecules. Such a single-molecule trap can strengthen CO 2 –host interactions without evoking chemical bonding, thus showing potential for CO 2 capture. Molecular single-molecule traps in the form of metal-organic polyhedra are designed, synthesised and tested for selective adsorption of CO 2 over N 2 and CH 4 , demonstrating the trapping effect. Building these pre-designed single-molecule traps into extended frameworks yields metal-organic frameworks with efficient mass transfer, whereas the CO 2 selective adsorption nature of single-molecule traps is preserved. Gas separation and purification are ongoing research topics, attracting interest from both academia and industry. In the last few years, CO 2 separation, as a key component of carbon capture, utilisation and storage, has become a fast-growing research area. Carbon capture, utilisation and storage may provide a temporary solution for the continued use of fossil fuels until renewable energy becomes abundant, alleviating the emission of anthropogenic greenhouse gases [1] , [2] . Two important clean-energy-related separations involving CO 2 are CO 2 capture from flue-gas streams of power plants, and natural-gas upgrading. The first entails separating CO 2 and N 2 , often under the harsh conditions of flue-gas streams from fossil-fuel-fired power plants. In natural-gas upgrading, from both natural reservoirs and landfills, the separation of CO 2 from CH 4 improves CH 4 purity and reduces pipeline corrosion by the acidic CO 2 gas. Various technologies for CO 2 capture/separation from its mixture with other gases have been developed, including the relatively mature amine-scrubbing procedure [3] , and other techniques that are under intense exploration. Among them, adsorptive and membrane-based separations are some of the most promising because of their potential for simple and low-energy-consumption processes. The performance of porous materials, the supporting medium of adsorbent and membrane, is critical for efficient separation. Many porous solids such as zeolites and activated carbons have been widely studied for clean-energy-related separations, including CO 2 capture [4] . However, methods for precise structural and property control of these materials, particularly at the molecular level, are still lacking. Recently, remarkable progress has been made in this regard in the development of metal-organic materials (MOMs), such as metal-organic frameworks (MOFs) [5] , [6] and metal-organic polyhedra (MOPs) [7] , assembled from molecular building units. These materials possess unique properties and vast application potential [8] , [9] , [10] , [11] , [12] , [13] , [14] , [15] , [16] , [17] , [18] , [19] , [20] , [21] , [22] , [23] , [24] . The hallmark of these new materials is their modular design, which is far beyond the scope of other porous materials [22] , [25] , [26] , [27] , [28] , [29] , [30] , [31] , [32] , [33] , [34] , [35] , [36] and allows for facile structure and property tuning. This therefore enables precise control of functions by accurate design of structures at the molecular level. Although many MOFs have been prepared for CO 2 separation in recent years, a precise construction implemented at the true molecular level is rare. Herein, as an experimental proof-of-concept, we demonstrate how it is possible to design a cavity specifically for the capture of a single CO 2 molecule. The first step is the design and synthesis of a molecular cavity, designated ‘single-molecule trap’ (SMT) for the convenience of discussion, starting from the evaluation of the size and properties of the guest CO 2 molecule ( Fig. 1a ). As molecular building blocks, these SMTs can be linked to construct a three-dimensional (3D) MOF to ensure efficient transport of CO 2 in and out of the cavities. 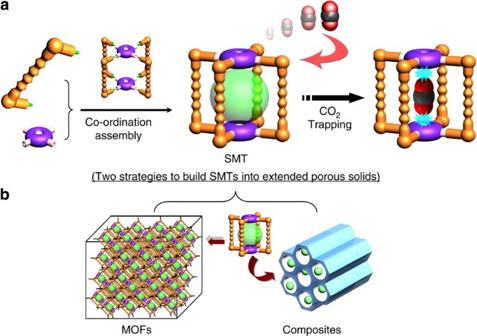Figure 1: Designing porous materials with SMTs for CO2molecule capture. (a) Schematic representation of the design and construction of a SMT for CO2adsorption. Organic linker is shown in orange, and the metal node with an open adsorption site is shown in purple and yellow; green spheres represent the cavity for CO2adsorption. (b) Two proposed strategies for building a pre-designed SMT into extended porous solids: assembly of the SMTs by ligand extension and accommodation of SMTs into other porous materials, such as mesoporous silica. An alternative route is the impregnation of an existing porous material such as mesoporous silica with SMTs directly ( Fig 1b ). In both cases, the selectivity of the SMT for CO 2 should be preserved. Figure 1: Designing porous materials with SMTs for CO 2 molecule capture. ( a ) Schematic representation of the design and construction of a SMT for CO 2 adsorption. Organic linker is shown in orange, and the metal node with an open adsorption site is shown in purple and yellow; green spheres represent the cavity for CO 2 adsorption. ( b ) Two proposed strategies for building a pre-designed SMT into extended porous solids: assembly of the SMTs by ligand extension and accommodation of SMTs into other porous materials, such as mesoporous silica. Full size image A CO 2 molecule is linear, about 2.4 Å long, positively charged at the C atom, and negatively charged at the O atoms. The normal M–O co-ordination bond length, where M represents a transition metal, is about 2.0–2.8 Å. Derived from the above distances, two positively charged ‘anchors’ [13] separated by about 6.4–8.0 Å (2.4+2 × M–O) distance would be ideal for holding a CO 2 molecule between them through electrostatic interactions. Negatively charged groups surrounding the C atom should strengthen the CO 2 –trap interaction even further. With these considerations in mind, we have prepared a molecular cage using four bridging ligands and two metal clusters (with open metal sites), which are separated by about 7.4 Å (from crystal structural determination) and expected to form strong electrostatic interactions with the negative O atoms of CO 2 , without the formation of a chemical bond. Such precisely designed SMTs should hold one CO 2 molecule per cavity, excluding other small molecules such as N 2 and CH 4 , allowing for the highly selective adsorption of CO 2 over other gases. Herein, we describe the design and synthesis of such functional porous materials for efficient CO 2 molecule capture, as well as the evaluation of the resulting materials by both molecular simulations and experiments. This exemplifies a new strategy in the highly controllable design and preparation of porous materials for specific adsorption-related applications. MOP-based SMTs for CO 2 selective adsorption To construct a MOP with fixed shape and distance between metal atoms, an organic ligand with appropriate geometry and size is a prerequisite. Our recent success in the assembly of MOPs with a variety of shapes, sizes and functional groups, by tuning the bridging ligands, enables us to synthesise a single cavity specifically designed for the accommodation of one CO 2 molecule [7] , [37] . In this work, two dicarboxylic acid ligands, 3,3′-(naphthalene-2,7-diyl)dibenzoic acid ( H 2 L 1 ) and 3,3′-(1,8-naphthyridine-2,7-diyl)dibenzoic acid ( H 2 L 2 ) were designed and synthesised by Pd-catalysed coupling reactions between 3-(methoxycarbo nylphenyl)boronic acid and 2,7-dibromonaphthalene or 2,7-dibromo-1,8-naphthyridine, respectively, followed by hydrolysis of the corresponding esters. With the ‘ cis and parallel’ arrangement of the two carboxylic acid groups in each ligand, both have a bridging angle of 0° and an inter-carboxylic-acid distance of about 7 Å, thus fulfilling both metal–metal distance and anchor orientation requirements in the resulting MOPs. The SMTs were assembled from H 2 L 1 and H 2 L 2 , shown in Fig. 2a , by reacting with Cu 2 (OAc) 4 ·2 H 2 O in N , N -dimethylacetamide (DMA) to give isostructural [Cu 2 ( L 1 ) 2 (DMA) 2 ] 2 ( SMT-1 -DMA) and [Cu 2 ( L 2 ) 2 (DMA) 2 ] 2 ( SMT-2 -DMA), at room temperature as phase-pure crystals, confirmed by a good match between the experimental and simulated powder X-ray diffraction (PXRD) patterns ( Supplementary Figs S1 and S2 ). 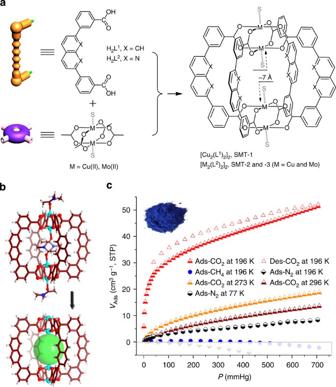Figure 2: Synthesis, structures and CO2selective adsorption of precisely designed SMTs. (a) Schematic representation of the construction ofSMT-1–3:Sis the coordinated solvent molecule, which can be removed through sample activation to yield an empty molecular cage for gas adsorption. (b) The molecular structure ofSMT-1with (top) and without (bottom) coordinated solvent molecules. The colour schemes: Cu, cyan; O, red; N, blue; C, brown; and H, light grey. The green sphere represents the free space inside the molecular cage. (c) Gas adsorption isotherms ofSMT-1, showing selective adsorption of CO2over CH4and N2(inset: a picture of activatedSMT-1sample). Figure 2: Synthesis, structures and CO 2 selective adsorption of precisely designed SMTs. ( a ) Schematic representation of the construction of SMT-1–3 : S is the coordinated solvent molecule, which can be removed through sample activation to yield an empty molecular cage for gas adsorption. ( b ) The molecular structure of SMT-1 with (top) and without (bottom) coordinated solvent molecules. The colour schemes: Cu, cyan; O, red; N, blue; C, brown; and H, light grey. The green sphere represents the free space inside the molecular cage. ( c ) Gas adsorption isotherms of SMT-1 , showing selective adsorption of CO 2 over CH 4 and N 2 (inset: a picture of activated SMT-1 sample). Full size image The structures of the two compounds were determined by single crystal X-ray diffraction. As expected, both MOP molecules have a lantern-type structural arrangement with four bridging ligands surrounding two paddlewheel dicopper motifs to form a large paddlewheel tetragonal cage ( Fig. 2b and Supplementary Figs S13 and S14 ). Each copper atom is coordinated by four carboxylate oxygen atoms of different ligands in the equatorial positions and one DMA molecule in the axial position, which can be removed to leave an open metal site. The dimensions of the two MOPs excluding coordinated solvents in height (Cu–Cu) and diameter (C–C between two opposite ligands) are 12.6 × 19.4 and 11.9 × 19.8 Å, respectively; and the inner cavity sizes are 7.4 × 10.7 and 6.7 × 12.5 Å (atom-to-atom distances across opposite Cu and H (or N ) atoms of ligands). Particularly, the distances between two opposite copper sites in each cavity of SMT-1 and -2 are 7.4 and 6.7 Å, respectively, suitable for the accommodation of one CO 2 molecule through the interaction of its two O atoms to the copper sites. Similarly, the reaction between H 2 L 2 and Mo 2 (O 2 CCF 3 ) 4 afforded compound [Mo 2 ( L 2 ) 2 (DMA)] 2 ·2DMA ( SMT-3 -DMA), with a similar structure to that of SMT-2 -DMA (see Supplementary Fig. S15 ). The size of the molecule and dimensions of the cavity are 11.5 × 20.3 and 7.3 × 12.9 Å, respectively. The methanol-exchanged SMT-1 -DMA was further activated under a vacuum at 80 °C to give desolvated material, SMT-1 , which, as a representative of these SMTs, was tested for gas adsorption. As shown in Fig. 2c , SMT-1 shows a significant adsorption for CO 2 at both low and enhanced temperatures, but almost excludes N 2 and CH 4 . At 196 K and 1 atm, the uptake of CO 2 is 52 cm 3 g −1 (2.32 mmol g −1 ), corresponding to about 4 CO 2 molecules adsorbed per SMT-1 molecule, implying that besides the cavities of SMT molecules, the space between them are also accessible for CO 2 adsorption. The evaluated Langmuir surface area is 153.7 m 2 g −1 and the pore volume is 0.097 cm 3 g −1 , based on the CO 2 adsorption data at 196 K. The adsorption capacity of CO 2 at 273 and 296 K are 19 (0.85) and 14 (0.63) cm 3 g −1 (mmol g −1 ), corresponding to about 1.5 and 1 CO 2 molecules per SMT-1 , respectively. The CO 2 adsorption enthalpy at zero coverage is ca. −35 kJ mol −1 (see Supplementary Fig. S17 ), higher than that in most MOFs, particularly those constructed from pure carboxylate ligands and similar paddlewheel dicopper clusters [5] , [38] . However, at 196 K and higher temperatures, the adsorption of N 2 and CH 4 falls below the detection limit of our instrument. The lack of accurate data sets for N 2 and CH 4 adsorption limits the quantitative estimation of adsorption selectivities of these gases in this porous molecular material. It should also be pointed out that the desolvated SMT-1 sample is still crystalline, as confirmed by PXRD ( Supplementary Fig. S1 ), but the diffraction peaks deviate from those of fresh SMT-1 -DMA due to the axial ligand removal and the resulting overall parking structure distortion. This observation differs from those of several previously reported MOP materials, which usually became amorphous after the solvent molecules were removed, but are still porous at the molecular level [7] , [37] . In addition, SMT-2 also adsorbs CO 2 up to 25 cm 3 g −1 (1.11 mmol g −1 ) at 273 K, but the uptakes of N 2 and CH 4 are well below the detection limit (see Supplementary Fig. S18 ). It is clear that these precisely designed SMTs are efficient for the selective CO 2 adsorption. To evaluate whether the CO 2 molecule prefers staying in the cavity of these SMTs, the CO 2 -binding energy of the SMTs with a variety of proposed metal sites (Zn, Cu, Rh and Mo) was calculated using density functional theory (DFT). The simulation indicates that it is indeed energetically favourable for a CO 2 molecule to stay in the cavity of these SMTs (see Supplementary Table S9 ). Moreover, SMTs with different metal ions show distinct affinities towards CO 2 . Among them, the Zn-based SMT shows the strongest interaction with a trapped CO 2 molecule, and the Mo-based one exhibits the weakest CO 2 affinity. These different CO 2 affinities arise from the ligand field preference of the metal ions. For example, the Mo 2 4+ cluster contains a quadruple bond and usually interacts weakly with axial ligands/guests [37] . The Zn-containing paddlewheel unit, on the other hand, contains no metal–metal bond. After removal of the coordinated solvent molecules, each Zn 2+ ion in the simulated compound prefers penta-coordination to square-pyramidal ligand environment through accepting an additional coordinating guest (such as CO 2 ), or to transfer to a tetrahedral environment. Because of the instability of square planar Zn 2+ , it is difficult to synthesise robust Zn-based SMTs, or other MOFs built from Zn-based paddlewheel units. The overall valid porosity of a MOP in the bulk sample is usually discounted because of the partial conglomeration of individual cages. When incorporated into a rigid porous framework, much more internal surface of MOP cages should become accessible. Building the pre-designed SMTs into extended materials Success in the construction of SMTs and their efficient capture of CO 2 molecules motivated us to build these molecular cages into extended framework materials to fully expose their internal surface and efficiently enhance the mass transfer for CO 2 adsorption and separation. The two above-mentioned strategies shown in Fig. 1 were tried initially, but only one, introducing the SMTs as building units into a MOF, has thus far been achieved. Incorporating these SMTs into other porous materials was hampered by the poor solubility of them in all tested solvents. To avoid precipitation of the SMT intermediate, we designed a ligand with two types of carboxylate groups, one to support the SMT and the other for the formation of an extended framework. Thus, an extended framework with SMTs can be assembled in a one-pot reaction. 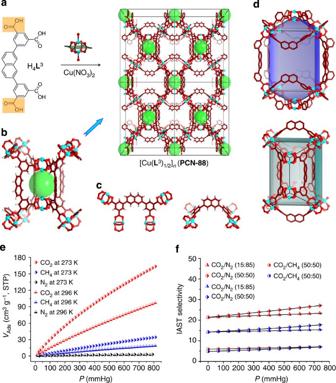Figure 3: Construction, structure and selective gas adsorption performance of a MOF with built-in pre-designed SMTs. (a) Schematic representation of the construction ofPCN-88and its 3D framework structure. Colour scheme: Cu, cyan; O, red; C, brown; and H, light grey. The green sphere represents the free space inside the built-in SMTs. (b) A SMT unit inPCN-88with its linkages towards extending to the 3D framework. (c) Two conformers of ligandL3observed inPCN-88. (d) Two complementary polyhedra (elongated convex/concave square dipyramid) inPCN-88structure. Each polyhedron is formed by connecting dicopper nodes as vertices. (e) CO2, CH4and N2adsorption isotherms ofPCN-88at two temperatures. (f) Pressure-dependent IAST adsorption selectivities of CO2over N2and CH4at 273 K (red) and 296 K (blue) inPCN-88calculated based on single-component adsorption data. In this context, the dicarboxylic acid ligand H 2 L 1 was functionalised by adding two additional carboxylic acid groups to generate 5,5′-(naphthalene-2,7-diyl)diisophthalic acid ( H 4 L 3 , Fig 3a ), which was synthesised by a procedure similar to that of H 2 L 1 , with diethyl 5-(4,4,5,5-tetramethyl-1,3,2-dioxaborolan- 2-yl)isophthalate instead of 3-(methoxycarbonylphenyl)boronic acid. H 4 L 3 reacted with Cu(NO 3 ) 2 ·2.5 H 2 O under solvothermal conditions (85 °C for 2 days) affording [Cu( L 3 ) 1/2 ( S )] n ( PCN-88 - S ) (porous coordination network (PCN), S represents non-assignable solvent molecules), which has a 3D framework structure containing the pre-designed SMT-1 units. The phase purity of the product was confirmed by PXRD ( Supplementary Fig. S4 ) and the structure was analysed by single crystal X-ray diffraction (see Supplementary Information ). Figure 3: Construction, structure and selective gas adsorption performance of a MOF with built-in pre-designed SMTs. ( a ) Schematic representation of the construction of PCN-88 and its 3D framework structure. Colour scheme: Cu, cyan; O, red; C, brown; and H, light grey. The green sphere represents the free space inside the built-in SMTs. ( b ) A SMT unit in PCN-88 with its linkages towards extending to the 3D framework. ( c ) Two conformers of ligand L 3 observed in PCN-88 . ( d ) Two complementary polyhedra (elongated convex/concave square dipyramid) in PCN-88 structure. Each polyhedron is formed by connecting dicopper nodes as vertices. ( e ) CO 2 , CH 4 and N 2 adsorption isotherms of PCN-88 at two temperatures. ( f ) Pressure-dependent IAST adsorption selectivities of CO 2 over N 2 and CH 4 at 273 K (red) and 296 K (blue) in PCN-88 calculated based on single-component adsorption data. Full size image As shown in Fig. 3c , in PCN-88 , there exist two conformers of L 3 ligands, one ( α -) with a dihedral angle of approximately 90° between the central and peripheral rings, whereas the other ( β -) has a dihedral angle of approximately 0°, similar to a previously reported series [39] . In the MOF, four α - L 3 ligands bridge two dicopper paddlewheel motifs to form a lantern-type unit similar to SMT-1 , with eight additional carboxylate groups pointing to eight vertices of a quadrangular prism containing a SMT unit, in which the distance between two opposite copper sites in the cavity is about 7.4 Å ( Fig 3b ). Through these carboxylate groups, each quadrangular prism is linked to eight others by sharing eight dicopper motifs to form a 3D network ( Fig 3a ). In each end of a quadrangular prism, one of the four ‘blades’ of each of the four dicopper paddlewheel motifs are further capped by carboxylate groups of one β - L 3 ligand. On the other hand, only two types of supramolecular building units exist if the centres of all dicopper paddlewheel motifs are connected. One is shown in Fig. 3d , top, which is an elongated square dipyramid; the other is a concave elongated square dipyramid with the two pyramids inverted ( Fig. 3d , bottom). The two units are complementary to each other in space filling. Six units of one type surround one unit of the other octahedrally forming a 3D network. After removal of coordinated solvent molecules, the solvent-accessible volume of the crystal (13667.3 Å 3 out of the 18544.0 Å 3 per unit cell) is 73.7% (ref. 40 ). After activation of the as-synthesised material by successive methanol/dichloromethane solvent exchanges and heating at 100 °C under reduced pressure, PCN-88 retained its crystallinity as confirmed by PXRD ( Supplementary Fig. S4 ). N 2 and Ar adsorption isotherms at 77 and 87 K of the activated sample (see Supplementary Figs S19 and S21 , respectively) further revealed permanent porosity. A two-step adsorption was observed in N 2 and Ar isotherms, with Brunauer-Emmett-Teller (BET) and Langmuir surface areas of 3308 and 3845, m 2 g −1 , respectively, based on the N 2 adsorption data (calculated from the first step of the adsorption isotherm). The stepwise adsorption isotherm can be explained by the existence of both meso- and micro-porous cages in the structure, as observed previously in similar systems [15] . As shown in Fig. 3e , PCN-88 has a significant CO 2 (160 (7.14) and 94 (4.20) cm 3 g −1 (mmol g −1 )) uptake, but little CH 4 (33 and 18 cm 3 g −1 ) and N 2 uptake (2.6 and 2.1 cm 3 g −1 ) at 273 and 296 K and 1 atm, respectively. It should be pointed out that the CO 2 uptake capacity of PCN-88 at 296 K and 1 atm ranks among the highest for MOFs constructed from pure carboxylate ligands (see Supplementary Table S10 ) excluding the MOF-74 series, which are constructed from ligands with –OH moieties [5] , [38] . These observed selective adsorptions of CO 2 over CH 4 and N 2 can be attributed to the much stronger interactions of the CO 2 molecule with the adsorbent surface compared with those of the other two gases. The calculated Henry’s law selectivities of CO 2 /CH 4 and CO 2 /N 2 are 7.3 and 67.9 at 273 K, and 5.3 and 18.1 at 296 K, respectively. Furthermore, ideal adsorbed solution theory (IAST (ref. 41 ) selectivities are also calculated by using the adsorption data of single-component gases ( Fig. 3f ). The values of IAST selectivities at 273 K and 1 bar for a 15/85 and a 50/50 CO 2 /N 2 mixture are 23.1 and 27.4, respectively; and those at 296 K and 1 bar are 15.2 and 17.6, respectively. For a 50/50 CO 2 /CH 4 mixture, corresponding values are 7.1 at 273 K and 7.0 at 296 K and 1 atm. The highly selective adsorption of CO 2 over N 2 and CH 4 suggests possible application of PCN-88 in capturing CO 2 from flue gas or upgrading natural gas. The zero-coverage heat of adsorption of CO 2 in PCN-88 is ca. −27 kJ mol −1 , which is higher than that in most MOFs constructed from pure carboxylate ligands and paddlewheel dicopper clusters [5] , [38] . This intermediate adsorption enthalpy implies a low-energy consumption for adsorbent regeneration, a desired property for separation applications. In fact, CO 2 capture in industry is highly process dependent, in which adsorbents are always optimised for a specific system. These equilibrium adsorption data only provide an initial step for improving the efficiency of a process. Additional experiments are still required for validating the practical value of these new adsorbents. The CO 2 , CH 4 and N 2 adsorption in PCN-88 have also been evaluated by grand canonical Monte Carlo (GCMC) simulations. The simulated adsorption isotherms of single-component gases closely match the experimental ones as shown in Supplementary Fig. S36 . To understand the adsorption behaviours of these gases in PCN-88 at the molecular level, snapshots of the structures with adsorbed gas molecules at 296 K and 1 atm were analysed (see Supplementary Fig. S37 ). It was found that the most preferred sites for CO 2 adsorption in PCN-88 are the corner regions close to metal sites, probably because of the strong electrostatic interaction between them. On the contrary, CH 4 and N 2 molecules prefer to be adsorbed around the organic units because of van der Waals interactions. Furthermore, the adsorption behaviours and selectivities of gas mixture containing 15% CO 2 and 85% N 2 (mimicking real flue gas), as well as 50% CO 2 and 50% CH 4 in PCN-88 , at different temperatures were also evaluated with GCMC simulations; the results are shown in Supplementary Figs S38–40 . The evaluated adsorption selectivity of CO 2 over N 2 is about 15.3 and 10.2, and for CO 2 over CH 4 is 5.2 and 3.8 at 273 and 296 K and 1 atm, respectively. It is much more interesting that the snapshot at 296 K for the CO 2 /N 2 mixture adsorption in PCN-88 shows that there are quite a few CO 2 molecules but no N 2 molecules absorbed in the trap cavities. In some cases, the CO 2 molecule actually ‘stands up’ in the trap cavity, as shown in Fig. 4 , demonstrating the validity of this designed SMT for CO 2 selective capture. 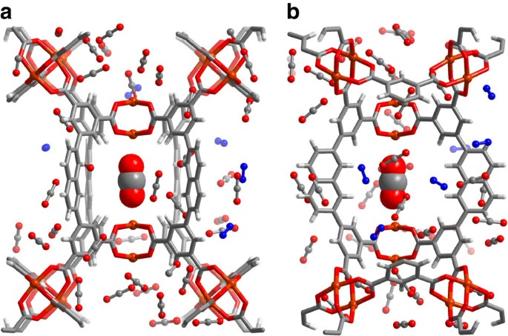Figure 4: Simulated locations of CO2and N2molecules in PCN-88 for CO2/N2(15:85) mixture. Simulation performed with a CO2/N2(15:85) mixture at 296 K and 3 Mpa. Viewed from different directions: (a) along the crystallographiczdirection and (b) along thexdirection. Colour scheme: Cu, dark orange; O, red; N, blue; C, dark grey; and H, light grey. It is clear that one CO2molecule (shown in space-filling model) can be trapped in the centre of a SMT cavity. Figure 4: Simulated locations of CO 2 and N 2 molecules in PCN-88 for CO 2 /N 2 (15:85) mixture. Simulation performed with a CO 2 /N 2 (15:85) mixture at 296 K and 3 Mpa. Viewed from different directions: ( a ) along the crystallographic z direction and ( b ) along the x direction. Colour scheme: Cu, dark orange; O, red; N, blue; C, dark grey; and H, light grey. It is clear that one CO 2 molecule (shown in space-filling model) can be trapped in the centre of a SMT cavity. Full size image In addition, the diffusion of CO 2 and its mixture with N 2 in PCN-88 at 296 K has also been studied by molecular dynamic simulations (see Supplementary Figs S43 and S44 ). It was found that single CO 2 molecules can diffuse into trap cavities but cannot be trapped at low loading; however, with increased loading, CO 2 is trapped in the cavities. For CO 2 /N 2 mixtures, it was confirmed that only CO 2 molecules can be trapped in the cavities, which is consistent with the GCMC simulations discussed above. Again, this result shows that the pre-designed SMTs in PCN-88 work well in selectively capturing CO 2 molecules. SMT’s impact on CO 2 adsorption in PCN-88 To further evaluate the effect of the SMTs on CO 2 adsorption in PCN-88 , a control experiment was designed and performed. As shown in Fig. 5a , blocking the cavities of SMTs in PCN-88 results in MOF [Cu( L 3 ) 1/2 (pyrazine) 1/12 ( S )] n ( PCN-88′ -S ), in which the trap cavities are occupied by pyrazine molecules by coordinating to two copper sites. PCN-88′ -S was synthesised by a one-pot reaction of H 4 L 3 , pyrazine and Cu(NO 3 ) 2 ·2.5 H 2 O under conditions similar to that for PCN-88- S . Its structure is almost identical with that of PCN-88- S except for the blocked SMTs as mentioned above. The structure contains a pore-accessible volume of 72.6% (13530.0 out of the 18646.0 Å 3 per unit cell volume) after removal of the coordinated solvent molecules [40] . The permanent porosity of desolvated material, PCN-88′ , was revealed by the N 2 and Ar adsorption (see Supplementary Figs S20 and S22 ) at 77 and 87 K, respectively. The evaluated BET and Langmuir surface areas are 3042 and 3799, m 2 g −1 , respectively, based on N 2 adsorption data. Similar to that of PCN-88 , two-step adsorption isotherms for N 2 and Ar, and different adsorption quantities of CO 2 (119 (5.31) and 70 (3.13) cm 3 g −1 (mmol g −1 )), CH 4 (27 and 15 cm 3 g −1 ) and N 2 (2.4 and 1.8 cm 3 g −1 ) at 1 atm and 273 and 296 K, respectively, were observed (see Supplementary Fig. S31 ). Clearly, compared with PCN-88 , PCN-88′ yields a lower adsorption capacity towards these gases at 273 and 296 K due to the blocked SMT cavities. Interestingly at 195 K, both MOFs show almost the same CO 2 uptake capacities of about 850 cm 3 g −1 at 1 atm; however, PCN-88 has a significantly enhanced CO 2 uptake compared with PCN-88′ at pressures below 0.60 atm (450 mmHg), particularly at about 0.20 atm (150 mmHg) ( Fig. 5c ). This much higher adsorption at low pressure (lower than 150 mmHg) may be attributed to the contribution from SMTs in PCN-88 , which is, as anticipated, very important for CO 2 separation from other gases, such as N 2 in flue gases, where the partial pressure of CO 2 is about 0.15 atm. For PCN-88′ , the calculated Henry’s law selectivities for CO 2 over CH 4 and N 2 are 6.1 and 49.4 at 273 K, and 5.0 and 12.6 at 296 K, respectively. Calculated IAST selectivities are 16.5 and 18.5 at 273 K and 1 bar, and 12.3 and 14.6 at 296 K, for 15/85 and 50/50 CO 2 /N 2 mixtures, respectively. The related values for a 50/50 CO 2 /CH 4 mixture are 6.6 and 5.8 at 273 and 296 K and 1 bar, respectively. All these evaluated selectivities in PCN-88′ are lower than those in PCN-88 (see Supplementary Table S6 ), indicating that the SMTs in the former have an effect on the selective adsorption of CO 2 over CH 4 and N 2 . The zero-coverage heat of adsorption of CO 2 in PCN-88′ is –25 kJ mol −1 , again lower than that in PCN-88 . In addition, it was also noted that PCN-88 has a higher H 2 uptake than that of PCN-88′ at 77 and 87 K, respectively, but both show similar adsorption enthalpies (see Supplementary Figs S24–26 ). In conclusion, this control experiment shows that the pre-designed SMTs in PCN-88 have a significant influence on the adsorption of CO 2 in the low-pressure region. 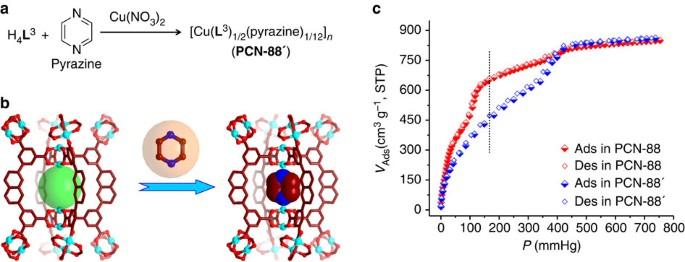Figure 5: Control experiment to identify the effect of SMTs in the PCN-88 on CO2adsorption. (a) Schematic representation of the synthesis ofPCN-88′. (b) Schematic representation of introducing a pyrazine molecule into the cavity ofPCN-88to block the SMT. Colour scheme: Cu, cyan; O, red; and C, brown. The green sphere represents the free space inside the SMT. (c) CO2adsorption isotherms ofPCN-88and -88′at 196 K, showing significantly different uptakes at low pressure due to the contribution of SMTs in the former. Figure 5: Control experiment to identify the effect of SMTs in the PCN-88 on CO 2 adsorption. ( a ) Schematic representation of the synthesis of PCN-88′ . ( b ) Schematic representation of introducing a pyrazine molecule into the cavity of PCN-88 to block the SMT. Colour scheme: Cu, cyan; O, red; and C, brown. The green sphere represents the free space inside the SMT. ( c ) CO 2 adsorption isotherms of PCN-88 and - 88′ at 196 K, showing significantly different uptakes at low pressure due to the contribution of SMTs in the former. Full size image All results discussed above evidently demonstrate the feasibility of precisely designing a cavity in porous MOMs for specific adsorption-based applications. Clearly, designing a MOF or other composite with a higher density of SMTs will substantially improve the overall adsorption performance of a particular guest molecule, such as CO 2 in this SMT-based system presented here. For many years, there has been a push towards porous materials with high surface areas and large pore sizes, particularly for MOFs. But for CO 2 selective adsorption or capture (also for H 2 storage), these features have not been effective. Recently, a strategy based on pore space partition in a MOF through cage-within-cage, or core-shell, type architecture has been proposed by Bu and colleagues [42] , as a strategy to optimise the pore space for better CO 2 capture. But the cage-within-cage configuration does not address the individual fit between the partitioned pore space and the size of the gas molecule. Here we represent the first time (to our knowledge) to design a cage-type assembly to specifically address the trapping of a particular molecule based on its chemical (polarity and so on) and physical (size and shape) properties. The advantage of this method is that it not only enhances the host–guest interactions because of an optimum fit, but it also simultaneously endows the material with superior selectivity over other guest molecules because the cavity is custom-designed for a specific molecule. In summary, a new concept, the ‘SMT’ has been utilised in designing porous materials at the molecular level for specific adsorption-based applications. As an experimental proof-of-concept, such a SMT was first designed and synthesised for CO 2 molecule capture by the precise selection of organic ligand and metal node to form a MOP. Experimental and computational simulation results demonstrate the efficiency of this MOP-based SMT in the preferential adsorption of CO 2 over N 2 and CH 4 , which are important for CO 2 capture from flue gas and CH 4 upgrading. Building this SMT into a MOF with an extended framework structure was achieved, again, through ligand design. This resulting MOF preserves the SMT properties in capturing CO 2 molecules, therefore showing good performance in the selective adsorption of CO 2 . In principle, by judiciously designing a SMT and thereby its extension into porous frameworks, this method can be applied in the synthesis of other new MOMs and composite materials for other specific applications, such as H 2 storage and even CO 2 activation by trapping one CO 2 in a confined cavity with strongly binding active sites. These materials may be used in applications such as small molecule capture, activation, conversion and storage, wherever binding single guest molecule is a prerequisite. Materials and syntheses All general reagents and solvents (analytical grade (AR) grade) were commercially available and used as received. The protonated ligands 3,3′-(naphthalene-2,7-diyl)dibenzoic acid ( H 2 L 1 ), 3,3′-(1,8-naphthyridine-2,7-diyl)dibenzoic acid ( H 2 L 2 ), 5,5′-(naphthalene-2,7-diyl)diisophthalic acid ( H 4 L 3 ) and 5,5′-(1,8-naphthyridine-2,7-diyl)diisophthalic acid ( H 4 L 4 , not used in the synthesis of MOFs because of its high cost) were newly designed and synthesised by using palladium-catalysed coupling reactions, followed by hydrolysis. The precursors in these reactions were purchased or synthesised according to the literature methods. SMT-1 -DMA and SMT-2 -DMA were synthesised by the reaction of Cu 2 (OAc) 4 ·2H 2 O with corresponding carboxylic acid ligands in DMA at room temperature. Single crystals of SMT-1 -DMA were obtained by layering a solution of H 2 L 1 in DMA upon a DMA solution of Cu 2 (OAc) 4 ·2H 2 O and staying for several days. For SMT-2 -DMA, two solutions of H 2 L 2 and Cu 2 (OAc) 4 ·2H 2 O in DMA were mixed and left undisturbed for several days to obtain crystals. Single crystals of SMT-3 -DMA were synthesised by heating a DMA solution of H 2 L 2 and Mo 2 (O 2 CCF 3 ) 4 with 48% aqueous solution of HBF 4 at 85 °C for 12 h. These SMT-DMA crystals slowly lose transparency as solvent molecules evaporate into the air over a longer period of time, and are insoluble in DMA, N,N -dimethylformamide, dimethyl sulfoxide, methanol and acetone. PCN-88- S and -88′- S were synthesised by similar solvothermal procedures: a DMA/water solution containing Cu(NO 3 ) 2 ·2.5H 2 O, H 4 L 3 ; a few drops of HBF 4 solution (and pyrazine for PCN-88′- S ) was heated at 85 °C for 2 days to afford single crystals. Phase purity of all products was evaluated by PXRD; general characterisation including infrared and thermogravimetric analysis were carried out. Detailed descriptions of syntheses and characterisation are given in the Supplementary Methods . X-ray single-crystal diffraction Data were collected on a Bruker AXS APEX-II CCD (charge-coupled device) diffractometer with a fine-focus sealed-tube X-ray source (Mo- K α ) and the structures were solved by direct methods. Details are provided in the Supplementary Information . In all the structures except SMT-3 -DMA, free solvent molecules are disordered, and attempts to locate and refine all the solvent molecule peaks were unsuccessful. Diffused electron densities resulting from these solvent molecules (except the O atoms of coordinated solvents) were removed from the data set using the SQUEEZE routine of PLATON and refined further using the data generated [40] . The coordinated solvent molecules in PCN-88- S and -88′- S are also disordered, only the O atoms were left and refined and other atoms were omitted. Contents of the removed solvent region are not represented in the unit cell contents in the crystal data of related compounds. Attempts to determine the final formula of these compounds from the SQUEEZE results, combined with elemental analysis and thermogravimetric analysis data, were unsuccessful because of the volatility of crystallisation solvents during measurements. Gas adsorption Gas adsorption measurements were performed using an ASAP 2020 volumetric adsorption analyser. A high-purity grade (99.999%) of gases was used throughout the adsorption experiments. Before adsorption, the sample was activated by solvent exchange (in several cycles using fresh methanol) to remove the coordinated DMA molecules, followed by degassing at elevated temperature and vacuum. Details are given in the Supplementary Information . To get more precise adsorption data, particularly for N 2 and CH 4 adsorption at higher temperatures, such as 296 K, the free space of the sample holder was minimised as much as possible. In evaluating the adsorption selectivities of these material towards different gases including CO 2 , N 2 and CH 4 , Henry’s law selectivity and IAST selectivity are calculated based on the adsorption data of each single gas. Computational simulations DFT calculations were performed for three purposes: to optimise the geometries of CO 2 interaction with SMTs; to evaluate the binding energies between CO 2 and SMTs; and to calculate the partial charges of PCN-88 framework atoms that were used in GCMC simulations. All DFT calculations were carried out using Gaussian 09 [43] . GCMC simulations were employed to calculate the uptake of single gases and gas mixtures in PCN-88, which was treated as a rigid framework, using the MUSIC program [44] . The potential parameters for the framework atoms were taken from DREIDING force field. Molecular dynamic simulations were performed using the DL-POLY-2.20 with the Berendsen thermostat in the NVT ensemble. Detailed descriptions and additional discussions are provided in the Supplementary Methods . Accession codes: The X-ray crystallographic coordinates for structures reported in this Article have been deposited at the Cambridge Crystallographic Data Centre (CCDC), under deposition number CCDC 867849 to 867853. These data can be obtained free of charge from The Cambridge Crystallographic Data Centre via www.ccdc.cam.ac.uk/data_request/cif . How to cite this article: Li J-R. et al . Porous materials with pre-designed single-molecule traps for CO 2 selective adsorption. Nat. Commun. 4:1538 doi: 10.1038/ncomms2552 (2013).